Neural organization of spoken language revealed by lesion–symptom mapping Studies of patients with acquired cognitive deficits following brain damage and studies using contemporary neuroimaging techniques form two distinct streams of research on the neural basis of cognition. In this study, we combine high-quality structural neuroimaging analysis techniques and extensive behavioural assessment of patients with persistent acquired language deficits to study the neural basis of language. Our results reveal two major divisions within the language system—meaning versus form and recognition versus production—and their instantiation in the brain. Phonological form deficits are associated with lesions in peri-Sylvian regions, whereas semantic production and recognition deficits are associated with damage to the left anterior temporal lobe and white matter connectivity with frontal cortex, respectively. These findings provide a novel synthesis of traditional and contemporary views of the cognitive and neural architecture of language processing, emphasizing dual routes for speech processing and convergence of white matter tracts for semantic control and/or integration. From the earliest days of cognitive neuroscience, detailed studies of patients with acquired cognitive deficits following brain damage have provided the strongest evidence regarding the neural basis of cognition. This is because focal brain injury can cause a specific and lasting impairment to a cognitive process only if the damaged region made an indispensable contribution to that process. Contemporary neuroimaging techniques permit investigators to study the neural basis of cognition and language with greater anatomical precision. The present study draws on the strengths of these distinct methods by combining broad and deep behavioural assessment, high-quality structural neuroimaging and contemporary neuroimaging analysis techniques, to examine the functional and neural organization of language processing in patients with acquired language deficits. The traditional neurological model of language and the brain [1] , [2] postulates a division between production and comprehension processes within the left peri-Sylvian cortex: lesions in posterior superior temporal regions (‘Wernicke’s area’) disrupt auditory language comprehension, lesions in inferior frontal regions (‘Broca’s area’) disrupt speech production and white matter lesions that disconnect these areas impair repetition of heard speech. Contemporary theories of language and the brain bear the important imprint of functional neuroimaging and they depart from the traditional view in important respects [3] . One proposal is that there are ‘primary’ brain systems for semantics, phonology and syntax, each contributing to both the comprehension and production of language [4] , [5] . Other ‘dual pathways’ models propose that language is subserved by two distinct pathways, differentially specialized for the recognition and production of speech [6] , [7] , [8] . Most contemporary models recognize the contribution of regions outside the classical peri-Sylvian language areas, particularly in relation to the processing of word and sentence meaning [9] , [10] , [11] , [12] . Finally, the advent of diffusion tensor imaging has led to an explosive growth in research on the fibre tracts of the brain and a re-evaluation of classical ‘disconnection’ accounts of aphasic and other syndromes [13] , [14] . The present study integrates several distinct threads of traditional and contemporary views by bringing together experimental psychology, cognitive neurology and neuroimaging methods. This study focuses on word-level language processing, because words are the primary building blocks of language—they form the critical junction point between the perceptual demands of speech recognition, the cognitive demands of processing meaning and the motor demands of speech production. Similar to the nineteenth century studies that produced the classical Broca–Wernicke–Lichtheim model, this study examined individuals with neurogenic language disorders, but on an unprecedented scale: 99 individuals with chronic language deficits (aphasia) following left hemisphere stroke were assessed on 17 different measures covering a wide range of language functions, including speech perception, spoken word production, verbal and non-verbal semantic cognition and short-term memory [15] . Factor analysis with varimax rotation was used to identify the key dimensions of variability in performance. This provided a data-driven model of the functional organization of language processing. Advances in neuroimaging analysis were then leveraged to carry out voxel-based lesion–symptom mapping (VLSM [16] ) and identify the brain regions where lesions produced deficits of these functional systems. See Methods section for a more detailed description of the participants, language tests and measures, and factor analysis and lesion analysis methods. The result is a novel synthesis that reveals two major divisions within the language system—meaning versus form and recognition versus production—and how they are instantiated in the brain. Factor analysis We used factor analysis with varimax rotation to identify key dimensions of variability on 17 measures of language function in 99 individuals with chronic language deficits following left hemisphere stroke. Three factors had eigenvalues above 1.0, passing the Kaiser threshold for inclusion in exploratory factor analysis. The first factor had high loadings from tests that require recognition of semantic relationships or matches, including verbal comprehension (word-to-picture matching and synonym judgments) and non-verbal comprehension (picture association judgments). These tests all require extracting task-appropriate semantic content from pictures or words but do not require substantial additional processing, as might be necessary for categorical inference or semantically driven word production; hence, we call this factor ‘Semantic Recognition’. The second factor had high positive loadings from tests of word and nonword repetition and negative loading from production of phonological errors in picture naming. These tests capture phonological/articulatory encoding for speech production; hence, we call this factor ‘Speech Production’. The third factor had high loadings from auditory lexical decision and phoneme discrimination tests, and moderate loadings from rhyme discrimination and word and nonword repetition tests. These tests capture auditory-phonological perception; hence, we call this factor ‘Speech Recognition’. The fourth factor had eigenvalue just below 1.0 (0.947), but had only one high loading: semantic errors in picture naming. Semantic error production was only moderately correlated with deficits on measures of semantic recognition (all Kendall rank correlations: τ <0.25) and, in a three-factor solution, this behavioural score did not load strongly on any of the factors (all loadings <0.4), suggesting that it is relatively independent of the other factors. Semantic errors in naming were previously analysed in a subset of the present group [17] , [18] and they provide a potentially important comparison for the first factor; thus, this factor was also retained (we will refer to it as ‘Semantic Errors’). The resulting four-factor solution captured 76% of the variance in the original data and the loadings are shown in Fig. 1 . 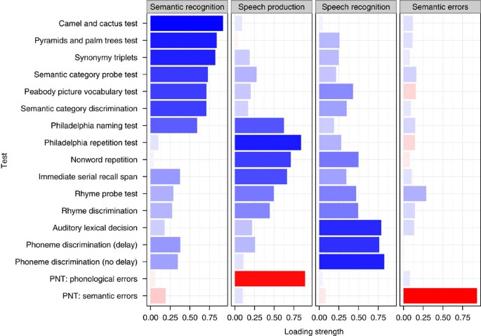Figure 1: Factor analysis results. Each panel shows the factor loadings of each test on the named factor. Longer and more saturated bars correspond to stronger loadings, with blue indicating positive loading and red indicating negative loading. See Methods for detailed descriptions of the tests and performance measures. Figure 1: Factor analysis results. Each panel shows the factor loadings of each test on the named factor. Longer and more saturated bars correspond to stronger loadings, with blue indicating positive loading and red indicating negative loading. See Methods for detailed descriptions of the tests and performance measures. Full size image The factor scores tended to be negatively correlated with lesion volume: larger lesions were associated with poorer performance on the Semantic Recognition factor (Kendall rank correlation: τ =−0.23, P <0.001), the Speech Production factor ( τ =−0.19, P <0.01) and the Semantic Errors factor ( τ =−0.18, P <0.01), although not on the Speech Recognition factor ( τ =−0.06, P >0.3). Therefore, the VLSM analyses included a control for lesion size that amounted to weighting lesioned voxels from small lesions more heavily than those from larger lesions (see Methods for details). The data-driven factor analysis approach revealed two major divisions in the cognitive architecture of language processing. The first was between semantic and phonological processing: in this large group of individuals with aphasia from left hemisphere stroke, the severity of deficits related to semantic processing varied independently from severity of deficits related to phonological processing. Both the semantic and phonological processing deficits could be further subdivided roughly between recognition and production: severity of semantic or phonological deficits in word production varied independently from severity of deficits in semantic or phonological recognition. We next investigated the neural organization of this cognitive architecture by examining which lesion locations were associated with variation along these cognitive dimensions. Voxel-based lesion–symptom mapping VLSM of the Semantic Errors factor ( Fig. 2 ) reproduced (with a larger sample of participants and transformed behavioural measure) our group’s previous findings that focal lesions of the left anterior temporal lobe (ATL) are associated with increased semantic errors in picture naming [17] , [18] (and a similar pattern is observed in progressive aphasia due to neurodegenerative disease [19] , [20] ). The behavioural dissociation of the Semantic Errors factor from the Semantic Recognition factor further indicates that the left ATL is specifically involved in semantically driven spoken word production. This result also shows that there was sufficient statistical power to detect lesion–symptom associations in the left ATL. Theories that emphasize the role of the ATL in modality-independent semantic processing [10] , [19] , [20] , [21] , [22] , [23] would predict this as the most probable location where lesions would cause deficits in Semantic Recognition. 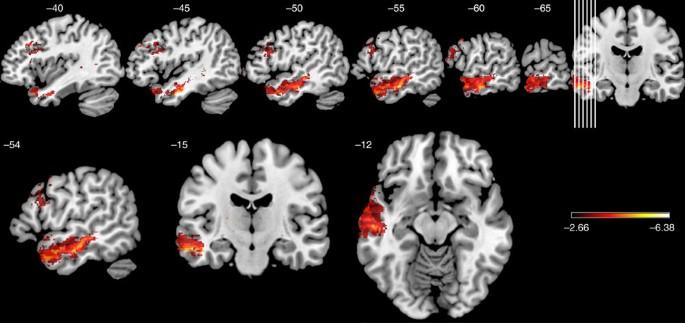Figure 2: VLSM of Semantic Errors. VLSMt-map supra-threshold (FDRq=0.05,t<−2.66) voxels for Semantic Errors factor scores with direct total lesion volume control. Figure 2: VLSM of Semantic Errors. VLSM t -map supra-threshold (FDR q =0.05, t <−2.66) voxels for Semantic Errors factor scores with direct total lesion volume control. Full size image VLSM of the Semantic Recognition factor identified no voxels in the ATL, even at a relaxed q =0.1 False Discovery Rate (FDR) threshold ( Fig. 3 ), nor were there voxels in any other cortical region typically associated with semantic processing, such as the middle temporal gyrus or the angular gyrus [9] , [24] . Instead, the identified voxels were primarily in the white matter medial to the insula and lateral to the basal ganglia. Several white matter tracts converge in this region, including the inferior fronto-occipital fasciculus, the uncinate fasciculus and the anterior thalamic radiations. The region did not include the superior longitudinal fasciculus (SLF III, which on some accounts corresponds to the fronto-parietal portion of the arcuate fasciculus [25] ): the SLF/AF passes dorsally to this region [26] or, on some accounts [27] , terminates posterior to it. The convergence of major white matter tracts in the identified area creates a ‘bottleneck’ where a small amount of damage can cause a large degree of dysfunction in connections between frontal cortices and the rest of the brain. The association with the semantic recognition factor probably owes to the fact that semantic cognition requires integration across multiple regions of a distributed cortical network [9] , [21] . Our proposal is that damage to the bottleneck region disrupts connectivity between the frontal lobe and other brain regions involved in semantic processing, consistent with other recent findings [28] , [29] , [30] . 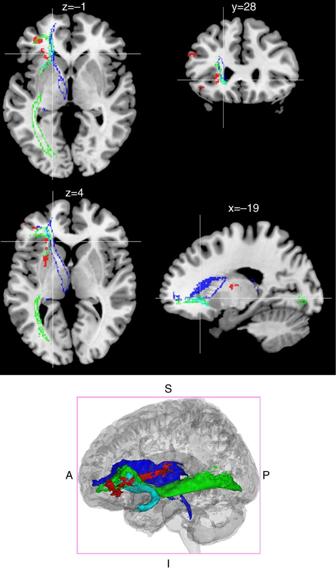Figure 3: VLSM of Semantic Recognition. VLSM of Semantic Recognition factor scores with direct total lesion volume control. Voxels exceeding FDR thresholdq=0.1 are shown in red, superimposed on outlines of key white matter tracts: uncinate fasciculus (light blue), inferior fronto-occipital fasciculus (green) and anterior thalamic radiations (blue). Bottom panel shows a tractography reconstruction of these tracts and the supra-threshold voxels using the same colour scheme. See Methods for details of white matter rendering. Figure 3: VLSM of Semantic Recognition. VLSM of Semantic Recognition factor scores with direct total lesion volume control. Voxels exceeding FDR threshold q =0.1 are shown in red, superimposed on outlines of key white matter tracts: uncinate fasciculus (light blue), inferior fronto-occipital fasciculus (green) and anterior thalamic radiations (blue). Bottom panel shows a tractography reconstruction of these tracts and the supra-threshold voxels using the same colour scheme. See Methods for details of white matter rendering. Full size image VLSM of the Speech Production factor identified a region superior to the Sylvian fissure, primarily in the supramarginal gyrus and extending anteriorly into inferior postcentral, precentral and premotor cortex ( Fig. 4 , blue–green). These regions form part of the dorsal language pathway of dual-pathway models and have been shown in other reports to be involved in speech production [6] , [31] , [32] . VLSM of the Speech Recognition factor identified a parallel region inferior to the Sylvian fissure, primarily in the superior temporal gyrus, including prominent involvement in Wernicke’s area and extending deep into planum temporale ( Fig. 4 , red–yellow). Together, these two factors map the classic peri-Sylvian language regions and the superior-inferior division between production and recognition provides new evidence to refine the dorsal–ventral division in dual-pathway models of speech processing [6] , [8] . 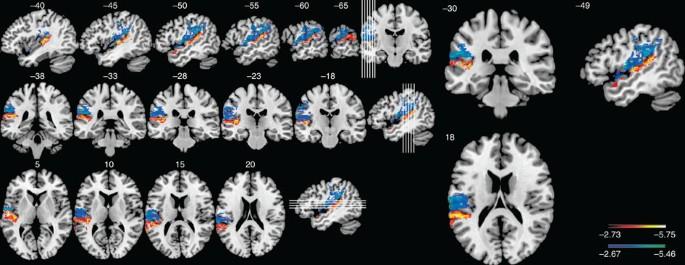Figure 4: VLSM of Speech Recognition and Production. VLSMt-map showing supra-threshold (FDRq=0.05) voxels for the Speech Production factor (blue–green) and the Speech Recognition factor (red–yellow) with direct total lesion volume control. Figure 4: VLSM of Speech Recognition and Production. VLSM t -map showing supra-threshold (FDR q =0.05) voxels for the Speech Production factor (blue–green) and the Speech Recognition factor (red–yellow) with direct total lesion volume control. Full size image By bringing together experimental psychology, cognitive neurology and neuroimaging methods, we have identified two divisions in the cognitive and neural organization of spoken language processing. The factor analysis results provide important new behavioural evidence of dissociation between semantic and phonological processes and between input and output processes. The first division corresponds to a set of peri-Sylvian regions for phonological processing and a separate set of extra-Sylvian regions for semantic processing. The peri-Sylvian regions involved in phonological processing were further subdivided into supra-Sylvian regions for speech production and infra-Sylvian regions for speech recognition. The extra-Sylvian regions involved in semantic processing were also divided between production and recognition processes. Impairment of semantic production, reflected in semantic errors, was strongly associated with left ATL lesions, whereas multimodal semantic recognition deficits were associated with impaired connectivity between the frontal lobe and other brain regions involved in semantic processing. The peri-Sylvian phonological processing regions were broadly consistent with dual-pathway models of speech processing [6] , [8] , [31] , [32] , [33] that propose a dorsal, temporal–parietal–frontal route for speech production and a ventral, temporal–frontal route for speech recognition and comprehension. Existing versions of this dual-stream framework differ in their claims regarding the anatomical structure of the streams, and the present data provide new insights to constrain these models. In the present study, the dorsal speech production route extends superior to the Sylvian fissure, from the supramarginal gyrus through inferior postcentral and precentral sensorimotor regions to premotor cortical regions involved in articulatory motor control. These results converge with previous findings implicating these areas in speech production tasks such as word repetition (after controlling for word recognition [31] , [33] , [34] ) and in the production of phonological errors in picture naming [32] . We did not find evidence to support the inclusion of inferior prefrontal cortex (Broca’s area), posterior planum temporale or posterior superior temporal gyrus (Wernicke’s area) in the dorsal speech production route. According to one influential dual-pathways model [6] , the dorsal stream, inclusive of these areas, subserves auditory-motor integration functions essential to speech production and some speech recognition tasks. Our findings support the involvement of planum temporale and Wernicke’s area in speech recognition, but as components of the ventral route, which our VLSM of Speech Recognition locates deep and inferior to the Sylvian fissure along the length of the superior temporal gyrus. This localization of the ventral route converges with a recent meta-analysis of functional neuroimaging studies that localized speech recognition processes to the superior temporal gyrus and revealed a posterior-to-anterior progression from recognition of speech sounds to spoken words in the superior temporal lobe [35] . The distinction between phonological input and output processes has been widely debated, often focusing on whether there are separate input and output lexicons [36] , [37] , and the roles of auditory speech codes in production [38] and articulatory motor codes in perception [39] , [40] . Although our results do not rule out the possibility that phonological input and output functions share certain codes or resources, they highlight the fact that extensive regions of peri-Sylvian cortex are differentially specialized for one or the other function. At the same time, our results demonstrate why a behavioural input–output dissociation would be difficult to observe. First, the factor analysis showed that many tasks involve both phonological input and output processes. For example, word and nonword repetition, immediate serial recall and rhyme discrimination all loaded on both the Speech Production and Speech Recognition factors, although to different extents. One of the virtues of factor analysis is that despite the fact that many tasks may involve multiple processes, factor analysis provides a data-driven way to identify an underlying structure and compute orthogonal performance measures on each dimension for each participant. Second, the VLSM showed that the regions involved in these processes are very close to one another; thus, it would be rare to find a patient with a lesion that only affected one neural substrate and not the other. Using VLSM with a large number of participants makes it possible to study lesion–symptom relationships at a finer neuroanatomical scale than would be possible with single-case or small group studies. The extra-Sylvian semantic processing regions also revealed a dissociation between semantically driven word production and recognition of semantic relationships in words and pictures, providing new insights into the architecture of semantic cognition. The Semantic Errors factor was associated with lesions in the ATL, consistent with other neuropsychological [17] , [19] , [20] and neuroimaging [41] findings that implicate this region in semantically driven retrieval of verbal labels. The ATLs have also been implicated in perceptual feature integration [42] and social semantic processing [43] . More relevant to the present study, it has been argued that the profile of multimodal semantic deficit observed in semantic dementia [10] , [19] , [44] originates from damage to ATL-localized ‘hubs’ in each hemisphere that integrate semantic information over the neurally distributed semantic network [9] , [10] , [21] . The behavioural and neural dissociation in the present data imposes some qualifications on this claim. The factor analysis revealed a very clear Semantic Recognition factor that combined verbal and non-verbal tests of recognition of semantic relationships or matches, similar to the multimodal semantic deficit in semantic dementia [10] , [19] , [44] . However, in this large group of left hemisphere stroke patients, this multimodal deficit was not associated with ATL lesions. As the production of semantic errors in picture naming was associated with ATL lesions, lack of lesion coverage in the ATL cannot explain our Semantic Recognition factor results. Rather, our results indicate that multimodal semantic deficits following unilateral left hemisphere stroke have a very different neuroanatomical basis [45] , [46] , [47] . Specifically, they arise from damage to a frontal white matter bottleneck—a region where the uncinate fasciculus, inferior fronto-occipital fasciculus and anterior thalamic radiations all converge. We suggest that this convergence produces a vulnerable location where a small amount of damage can have large functional consequences affecting semantic processing of both verbal and non-verbal (visual) input. Damage to this white matter bottleneck impairs connections between the inferior and middle portions of the frontal lobe and regions in the temporal, parietal and occipital lobes that are involved in semantic processing. Our results identify the importance of connections within the distributed semantic network but do not specify the role of those connections in semantic cognition. One possibility is that disruption of these connections impairs the multimodal integration critical for semantic cognition, similar to other disconnection-based accounts of cognitive deficits [13] , [14] . Another possibility, based on the role of the frontal regions in cognitive control [48] , [49] , is that the frontal lobes serve to shape or select semantic knowledge relevant for a given task and disruption of these connections impairs semantic control [45] , [46] , [47] . However, this account would have to explain why the critical region is in the deep white matter underlying the frontal lobe rather than in the (pre)frontal cortex itself. It is important to stress that these results are not inconsistent with findings from functional neuroimaging that a widespread bilateral cortical network is engaged by semantic processing tasks [9] , [21] , nor are our findings incompatible with evidence that lesions to other regions of the distributed cortical network are capable of producing semantic deficits [12] , [50] , [51] . Rather, building on evidence that semantic cognition is supported by a widely distributed neural system, our results emphasize the importance of white matter connections for integrating and/or selecting information across this network. Specifically, our results identify a region of fibre tract convergence where a small amount of damage can impair semantic processing across multiple tasks and modalities. Outside this bottleneck region, more extensive lesions would be required to produce comparable multimodal semantic deficits; small, focal lesions would be expected to produce deficits that are more domain specific. The behavioural dissociation of semantic errors from other measures of multimodal semantic processing has implications for cognitive models of word production, indicating that semantic errors in aphasic word production do not arise at the level of core semantic processing. Either they arise subsequent to semantic processing—in the mapping from semantics to lexical units [52] or in the mapping from semantics to phonology [53] —or they reflect damage to semantic processes specific to word production (that is, a modality-specific semantic deficit). In either case, our finding that lesions of the left ATL are associated with semantic errors, and not multimodal semantic deficits, provides new constraints on theories of the neural basis of semantic memory. First, the superior and middle portions of the left ATL appear to be specifically critical for semantically driven word retrieval—lesions here cause semantic errors in production but do not disrupt more general multimodal semantic processing. Second, semantic cognition (both semantic representation and semantic control) cannot be reduced to cortical hubs—the white matter connections play an integral role. Our evidence shows that a white matter lesion causes multimodal semantic deficits in stroke. In semantic dementia—the paradigmatic impairment of semantic representation—the ATL is frequently the site of peak grey matter atrophy, but the neurodegeneration extends beyond ATL, including into the fronto-temporal white matter, and recent evidence shows that this white matter degeneration also contributes to the semantic deficit [23] , [28] . We have emphasized the dissociation of semantic errors and multimodal semantic deficits, but our proposal does not require completely independent semantic systems for comprehension and production, only some functional specificity within the semantic system, such that different kinds of damage produce different kinds of deficits. Our proposal also explains why lesions in other regions known to be important for semantic processing, such as the middle and posterior portions of the middle temporal gyrus and the inferior parietal lobule (angular gyrus and supramarginal gyrus) [9] , [24] , [51] , [54] , were not associated with either semantic errors or multimodal semantics. Our data suggest that the role of these regions is neither specific to semantically driven word production (that role is played by the left ATL) nor general enough for focal damage to produce multimodal semantic deficits. In contrast, damage to the white matter bottleneck impairs connections among the widely distributed network of the left frontal–temporal–parietal regions involved in semantic cognition, thereby producing multimodal semantic deficits. The present study only included individuals with left hemisphere lesions; thus, it cannot speak to the possible hemispheric asymmetry between the ATLs, such that the left ATL is more strongly involved in verbal semantic tasks, whereas the right ATL is more involved in non-verbal (picture) semantic tasks [44] , [53] . In addition, as lesion coverage was poor in ventral and inferolateral temporal cortex, we cannot rule out bilaterally redundant multimodal semantic hubs in those sectors of the ATL [55] , but we can rule out damage to such hubs as an account of the multimodal semantic recognition deficit observed in aphasia following left hemisphere stroke. Finally, the present results do not identify critical sub-regions within the functionally and anatomically heterogeneous inferior and middle portions of the frontal lobe [56] , [57] . In conclusion, studies of patients with persistent cognitive deficits form the foundation of cognitive neuroscience, but such patients can be idiosyncratic and typically do not allow precise anatomical conclusions. Contemporary neuroimaging techniques offer a way to study the neural basis of cognitive processes on a wider scale and with finer anatomical precision, but it can be difficult to conclusively distinguish task-critical and ancillary neural (or hemodynamic) responses. The present study drew on the strengths of these distinct methods by combining broad and deep behavioural assessment of left hemisphere stroke patients with high-quality structural neuroimaging analysis techniques. The results reveal the functional and neural architecture of the language system with an unprecedented degree of neuroanatomical precision and offer a novel synthesis of the traditional separation of receptive and expressive language with the contemporary emphasis on primary systems. Participants Participants were drawn from an ongoing project investigating the anatomical basis of psycholinguistic deficits in post-acute aphasia. Results from this project and some of these participants have been reported in several previous publications [17] , [18] , [32] , [34] , [54] , [58] . In particular, the original demonstration that semantic errors in naming localize to the left ATL was based on 64 patients from the current group of 99 (refs 17 , 18 ). To be included in this study, participants had to be at least 1 month post onset of aphasia secondary to stroke, living at home, medically stable without major psychiatric or neurological co-morbidities and have been premorbidly right handed. Participants were also required to have English as the primary language, adequate vision and hearing (with or without correction) and computed tomography (CT) or magnetic resonance imaging (MRI) confirmed left hemisphere cortical lesion. Only participants who had completed all 17 tests were included in this study. All participants gave informed consent to take part in a multisession language assessment under protocols approved by the Institutional Review Boards at the Albert Einstein Medical Center and University of Pennsylvania School of Medicine. The sample consisted of 43 women and 56 men, 48 African Americans and 51 Caucasians. They averaged 58 years of age (s.d.=11; range=26–79), 14 years of education (s.d.=3; range=10–21) and 53 months post onset of stroke (s.d.=68; range=1–381). Eighty-three per cent were in the chronic phase (>6 months.) The predominant subtype diagnosis was anomic aphasia (44%), followed by Broca’s aphasia (27%) and conduction aphasia (16%). The Aphasia Quotient, which rates overall severity on a scale from 1 (most severe) to 100, averaged 73 (s.d.=18.4; range=27.2–97.9). Language tests Participants completed a multi-session battery of psycholinguistic tests, primarily focused on word-level processing, from speech perception to verbal and non-verbal semantic processing. Here we provide a brief description along with mean, s.d. and range of performance for each test. A more detailed description of the battery has been provided previously [15] . Camel and cactus test [59] : Test of non-verbal semantic processing in which a pictured item must be matched to the closest associate among a set of four pictured choices (for example, wine matched to: grapes, cherry, strawberry and orange). Performance is measured by per cent correct of 64 trials: M =75.2, s.d.=15.0, range=25–95. Pyramids and palm trees test [60] : Test of non-verbal semantic processing in which a pictured item must be matched to the closest associate among a set of two pictured choices (for example, fish matched to: cat and dog). Performance is measured by per cent correct of 52 trials: M =87.4, s.d.=11.5, range=46–100. Synonymy triplets [61] : Test of verbal semantic processing in which participants must decide which two of three words are most similar in meaning. Half the trials involve nouns (for example, violin, fiddle and clarinet), the other half verbs (for example, to repair, to design and to fix). Performance is measured by per cent correct of 30 trials: M =79.1, s.d.=16.9, range=33–100. Semantic category probe test [62] : Test of semantic short-term memory in which participants listen to a list of three or more words and must determine whether the final word is from the same category as any of the preceding words by saying or pointing to ‘Yes’ or ‘No’. The list of words gradually increases and performance is measured as the maximum list length with 75% or higher accuracy: M =2.18, s.d.=1.28, range=0.50–6.00. Peabody picture vocabulary test [63] : An untimed, norm-referenced spoken word-to-picture matching vocabulary test arranged in order of increasing difficulty and representing various parts of speech. Performance is measured by a standard score: M =79.9, s.d.=15.8, range=40–115. Semantic category discrimination (based on ref. 62 ): Test of verbal semantic processing in which participants must indicate whether two spoken words are members of the same semantic category by saying or pointing to ‘Yes’ or ‘No’. Performance is measured by per cent correct of 40 trials: M =82.9, s.d.=13.2, range=37–100. Philadelphia naming test [64] : A 175-item single-word picture naming test using black and white line drawings of minimal complexity and confusability. The target words cover a relatively wide range of word length, word frequency and semantic category. The pictures are all familiar objects with high name agreement (97% correct naming performance by unimpaired controls). Three performance measures were included: overall per cent correct ( M =63.3, s.d.=29.1, range=1.1–97.7), per cent of semantic errors (for example, naming elephant as zebra; M =5.4, s.d.=3.9, range=1.1–18.3) and per cent of phonological errors (for example, naming ghost as goath or horse as house; M =13.2, s.d.=13.3, range=0–49.1). Philadelphia repetition test : A word repetition test using the same set of 175 targets as the Philadelphia naming test. Performance is measured by per cent correct: M =85.9, s.d.=14.1, range=39–100. Nonword repetition : Pre-recorded nonword targets derived from Philadelphia naming test target words were presented to participants for repetition. Performance is measured by per cent correct of 60 trials: M =47.3, s.d.=25.8, range=0–98. Immediate serial recall span [65] : Test of short-term memory in which participants were required to repeat ten lists of one-syllable words, starting with two-word lists (‘wine–dream’) and increasing up to five-word lists, if possible (‘soul–fear–art–dream–shoe’). Performance is measured by span length of the form X . Y , where X is longest list that with at least 50% correct recall and Y is the proportion correct on the next list out of 50%: M =2.70, s.d.=1.09, range=0.50–5.00. Rhyme probe test [62] : Test of phonological short-term memory in which participants listen to a list of three or more words and must determine whether the final word rhymes with any of the preceding words by saying or pointing to ‘Yes’ or ‘No’. The list of words gradually increases and performance is measured as the maximum list length with 75% or higher accuracy: M =2.80, s.d.=1.69, range=0.50–7.31. Rhyme discrimination (based on ref. 62 ): Test of speech perception in which participants must indicate whether two spoken words rhyme by saying or pointing to ‘Yes’ or ‘No’. Performance is measured by per cent correct of 30 trials: M =88.7, s.d.=12.1, range=43–100. Auditory lexical decision (subtest of the psycholinguistic assessment of language processing in aphasia [66] ): Test of spoken word recognition in which participants must indicate whether each item is a real English word or not (80 items of each type). Performance is measured as overall d′ (a measure of discrimination based on signal detection theory): M =2.48, s.d.=0.70, range=0.33–3.88. Phoneme discrimination [61] : Test of speech perception in which participants must indicate whether two spoken words ( n =20) or nonwords ( n =20) are the same or different. Non-identical pairs differ by a single onset or final phoneme. In the delay version, there is a 5-s interval between the two items in a pair. Performance is measured by per cent correct. No delay: M =88.0, s.d.=11.6, range=48–100. Delay: M =81.6, s.d.=12.8, range=48–100. Factor analysis Performance of the 99 included participants on the 17 measures was subjected to principal components analysis with varimax rotation to produce orthogonal factors that, in the limit, would preserve all of the variance in the original data. The standard Kaiser criterion (extract factors with eigenvalue >1.0) was used to determine which factors captured meaningful variance in the data. This produced a three-factor model that captured 70% of the variance in the original data. The fourth factor consisted almost entirely of semantic errors, which did not load strongly on any of the three factors (all loadings <0.4) and the participants’ factor scores for the first three factors were virtually identical under the three-factor and four-factor models ( r >0.97 for each of the three factors). As these factor scores were the behavioural measures for the VLSM analyses, the three-factor and four-factor models would produce virtually identical VLSM results. We included this semantic errors factor in the analyses, because doing so would have virtually no impact on the other results and would be a useful comparison for factor 1 (Semantic Recognition) and with previous VLSM analyses of semantic errors. Lesion analysis Research brain scans were acquired for 87 participants (50 MRI and 37 CT). High-resolution whole-brain T1-weighted images (magnetization-prepared rapid acquisition gradient echo) were acquired for the 50 participants undergoing MRI. Of these, 44 were scanned on a 3-T Siemens Trio scanner (repetition time=1,620 ms, echo time=3.87 ms, field of view=192 × 256 mm, 1 × 1 × 1 mm 3 voxels). As medical implants were not approved for the higher strength magnetic field, six participants were scanned instead on a 1.5-T Siemens Sonata (repetition time=3,000 ms, echo time=3.54 ms, field of view=24 cm, 1.25 × 1.25 × 1.2-mm voxels). For 37 participants who were not eligible for MRI scanning, whole-brain CT scans without contrast (60 axial slices, 3 mm thick) were acquired. Twelve additional participants declined scanning; for these participants, recent clinical scans (CT ( n =8) and MRI ( n =4)) with clearly delineated lesion boundaries were substituted in the lesion tracing procedure. Lesions were manually segmented on the structural image by a trained technician or experienced neurologist, both of whom were blinded to the behavioural data. The lesion maps drawn by the technician were reviewed by the experienced neurologist. MRI structural scans were registered to a custom template constructed from images acquired on the same scanner and then from this intermediate template to the Montreal Neurological Institute space ‘Colin27’ volume. Lesions imaged with CT were drawn by the experienced neurologist directly onto the Colin27 volume, after rotating (pitch only) the template to approximate the slice plane of the patient’s scan (these procedures have been used in several previous studies [17] , [32] ). The lesion overlap map for the 99 qualified participants in the left hemisphere is shown in Supplementary Fig. 1 . Anatomical alignment of lesions does not guarantee functional alignment due to individual differences in functional organization and re-organization following stroke; however, large-scale studies such as this one provide the best evidence regarding aspects of functional organization that are consistent across individuals. VLSM analysis was performed for each factor. Only voxels lesioned in at least 10 participants were included in analysis, because tests of voxels where <10% of the participant sample has lesions would produce unacceptably unstable results. VLSM analysis was performed by running a simple regression analysis at each voxel, with the lesion status as the independent variable and the factor score as the dependent variable. To control the effect of total lesion volume, each lesion map was normalized to have a unit norm. After normalization, the lesion status of each subject equals either 0 (no lesion on this voxel) or the reciprocal of the norm of the lesion map, that is, 1/(square root of total lesion volume). This normalization process was adopted from a multivariate lesion–symptom mapping method [67] , where the lesion maps were normalized to have a norm of 1 to stabilize data processing. As total lesion volume is a big positive number, it is highly correlated to its square root ( r >0.99 for a random series); hence, the normalization is nearly the same as setting the lesion status to be 1/(total lesion volume). We call this approach ‘direct total lesion volume control’. After direct total lesion volume control, greater weight was placed on lesioned voxels when the total lesion volume was smaller than when it was larger. General linear model from SPM8 package ( www.fil.ion.ucl.ac.uk/spm/ , Wellcome Institute of Imaging Neuroscience, London, UK) was used to model the correlation between lesion status for each voxel and the factor scores. The general linear model coefficient β was used to measure the relative importance of each voxel to each factor. The VLSM β-values obtained from the genuine order of factor score were compared to those obtained by 1000 permutations of the factor score at each voxel, and the number of permutations yielding higher VLSM β-value than the genuine one was divided by 1001 to get the permutation p -value. The derived statistical p -map was thresholded with FDR q =0.05 (Semantic Recognition factor was thresholded with FDR q =0.1) and isolated clusters with voxel number no more than 50 after thresholding were removed. As a check, an alternative family-wise cluster correction method [68] was also used to determine a cluster size threshold by permuting the lesion–behaviour (factor score) relations (3,000 permutations), setting the voxelwise threshold to P <0.001 (uncorrected) and computing the minimum cluster size that would have a <5% likelihood of being exceeded by chance. This permutation-based family-wise cluster correction method produced the same pattern of results as the FDR correction; details of the method are provided in the Supplementary Methods along with figures showing the results ( Supplementary Figs 2–4 ). The white matter tracts in Fig. 3 were based on the ICBM-DTI white matter tractography atlas from FSL ( http://fsl.fmrib.ox.ac.uk/fsl/fslwiki/Atlases ) [27] , [69] , [70] using a 20% probability threshold. How to cite this article : Mirman, D. et al. Neural organization of spoken language revealed by lesion–symptom mapping. Nat. Commun. 6:6762 doi: 10.1038/ncomms7762 (2015).